Characterizing the genetic basis of innate immune response in TLR4-activated human monocytes Toll-like receptors (TLRs) play a key role in innate immunity. Apart from their function in host defense, dysregulation in TLR signalling can confer risk to autoimmune diseases, septic shock or cancer. Here we report genetic variants and transcripts that are active only during TLR signalling and contribute to interindividual differences in immune response. Comparing unstimulated versus TLR4-stimulated monocytes reveals 1,471 expression quantitative trait loci (eQTLs) that are unique to TLR4 stimulation. Among these we find functional SNPs for the expression of NEU4 , CCL14 , CBX3 and IRF5 on TLR4 activation. Furthermore, we show that SNPs conferring risk to primary biliary cirrhosis (PBC), inflammatory bowel disease (IBD) and celiac disease are immune response eQTLs for PDGFB and IL18R1 . Thus, PDGFB and IL18R1 represent plausible candidates for studying the pathophysiology of these disorders in the context of TLR4 activation. In summary, this study presents novel insights into the genetic basis of the innate immune response and exemplifies the value of eQTL studies in the context of exogenous cell stimulation. The innate immune system is the first line of defense against invading microorganisms. It is equipped with pattern recognition receptors (PRRs) that have evolved to sense conserved microbe-associated molecular patterns. Among other PRR families, Toll-like receptors (TLRs) play a pivotal role in antimicrobial defense, with TLR4 being one of the best-characterized member. TLR4 detects lipopolysaccharide (LPS) derived from Gram-negative bacteria and relays signal transduction to induce pro-inflammatory gene expression [1] . Apart from their antimicrobial function, TLRs also sense endogenous molecules, known as damage-associated molecular patterns [2] , [3] . Mutations and polymorphisms in TLR and TLR-signalling genes have been shown to confer susceptibility to many infectious and inflammatory diseases [4] , [5] . Here we perform transcriptome profiling in purified monocytes and genome-wide single-nucleotide polymorphism (SNP)-genotyping in 137 healthy individuals to identify transcripts and genetic variants that contribute to interindividual differences in TLR4 signalling. This innovative approach provides new insights into the genetic control of innate immune response. Expression profiling of unstimulated (baseline) and TLR4-stimulated monocytes revealed 9,031 differentially expressed transcripts at 90-min LPS exposure ( P <8.7 × 10 −07 , Bonferroni-corrected P value<0.01; Supplementary Fig. 1a ). A duration of 90 min was chosen to study a time point that covers the primary wave of gene expression (independent of de novo protein synthesis) with an informative set of differentially expressed genes following PRR stimulation [6] . Among the most strongly differentially expressed genes (mean log 2 fold change >1), pathway analyses revealed a significant enrichment of genes involved in PRR signalling and their respective outputs ( Supplementary Fig. 1b and Supplementary Data 1 ). Further subcategorization of differentially expressed genes into subsets of coexpressed genes allowed additional refinement of the ascribed signalling pathways to specific clusters ( Supplementary Fig. 1c and Supplementary Data 2 ). For both conditions—baseline and TLR4 signalling—expression quantitative trait loci (eQTL) analyses were performed and a false discovery rate (FDR) of 0.01 was used to define eQTLs ( P Baseline <8.67 × 10 −09 , P LPS <7.35 × 10 −09 ). To avoid underestimation of shared eQTLs between treated and untreated monocytes, we additionally conducted a multivariate analysis of variance (MANOVA) [7] ( P Manova <1.76 × 10 −09 , FDR-corrected P value<0.01, Supplementary Fig. 2a,b ). In addition, we calculated the differential expression of baseline vs TLR4-stimulated cells and performed eQTL analyses using an FDR of 0.01 ( P ΔLPS/Baseline <4.33 × 10 –10 ). In total, we identified 975 cis (corresponding to 292 genes) and 496 trans eQTLs (corresponding to 184 genes), which are unique to TLR4 stimulation ( Fig. 1b , Supplementary Fig. 3 ), as well as 435 cis (corresponding to 74 genes) and 17 trans eQTLs (corresponding to 8 genes), when differential expression (ΔLPS/Baseline) was considered ( Supplementary Fig. 4 ). A complete list of all significant eQTLs (baseline, LPS, ΔLPS/baseline) is provided by Supplementary Data 3–5 . 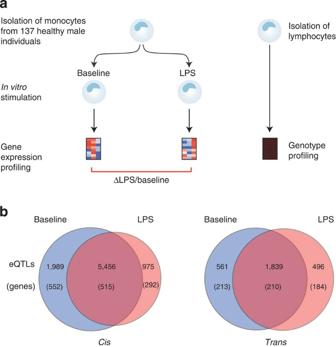Figure 1: Experimental design of the study in human monocytes of 137 healthy male donors. (a) Overview of step-wise study design applied in human monocytes. (b) Venn diagrams of eQTLs and corresponding transcripts of baseline (Baseline) and LPS-treated (LPS) monocytes incis(left) andtrans(right). Linear regression model was used for eQTL mapping. MANOVA was used to determine shared eQTLs. Figure 1: Experimental design of the study in human monocytes of 137 healthy male donors. ( a ) Overview of step-wise study design applied in human monocytes. ( b ) Venn diagrams of eQTLs and corresponding transcripts of baseline (Baseline) and LPS-treated (LPS) monocytes in cis (left) and trans (right). Linear regression model was used for eQTL mapping. MANOVA was used to determine shared eQTLs. Full size image Interestingly, analysing all eQTLs together (both cis and trans, baseline, LPS, ΔLPS/baseline) revealed a significant enrichment for lysosome-associated pathways, such as lysosomal enzymes and respective trafficking components ( Supplementary Fig. 5 , Supplementary Data 6 ). This is noteworthy, as lysosomes have been shown to play pivotal roles in both sensing and effector function of innate immune cells, our results suggest that there is a genetic contribution to these pathways [8] , [9] . In the following we focused on eQTLs unique to TLR4 signalling, both under absolute and differential expression, and refer to them as immune response eQTLs or iQTLs. In line with the pathway analysis above, our strongest iQTL ( Supplementary Table 1 ) is represented by the SNP rs3749155 on chromosome 2q37 and regulates the expression of neuraminidase 4 ( NEU4 ), which belongs to a group of lysosomal neuraminidases that catalyse the cleavage of sialic acids linked to glycoconjugates [10] . This iQTL is located in intron 3 of NEU4 and regulates its expression in cis ( P LPS =3.44 × 10 –44 , Fig. 2 ). In the context of innate immune signalling pathways, neuraminidases have been shown to regulate the activity of TLRs at the posttranslational level. For example, NEU1—the best-characterized neuraminidase—promotes the cleavage of sialic acids from the ectodomain of TLR4, which is a prerequisite for TLR activation [11] . Although a similar effect on TLR4 has been observed for NEU4 (ref. 12 ), the relevance of NEU4 to innate immunity has been less intensively studied so far. Our findings, however, suggest that genetic variability in NEU4 strongly contributes to interindividual differences in the innate immune response. 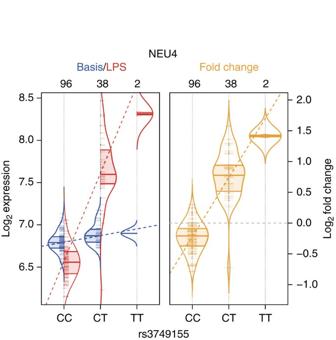Figure 2: rs3749155 represents the strongestcisiQTL during TLR4 signalling. Allele-specific gene expression in untreated versus LPS-treated monocytes is depicted as violin plots. The distribution of log2expression is shown on the left (blue: baseline, red: LPS) and log2fold change on the right (orange). The dashed lines indicate the regressions of the (Δ) gene expression values versus genotype. Individuals are indicated by small tick marks on the respective axes, with the group sizes per genotype indicated on top of each plot. The shaded ranges correspond to the 25–75% quartiles with the median indicated separately (analogous to a common boxplot). The violin plots show thatNEU4is induced in carriers of allele T on LPS exposure, whereasNEU4expression is reduced in homozygotes of allele C. Figure 2: rs3749155 represents the strongest cis iQTL during TLR4 signalling. Allele-specific gene expression in untreated versus LPS-treated monocytes is depicted as violin plots. The distribution of log 2 expression is shown on the left (blue: baseline, red: LPS) and log 2 fold change on the right (orange). The dashed lines indicate the regressions of the (Δ) gene expression values versus genotype. Individuals are indicated by small tick marks on the respective axes, with the group sizes per genotype indicated on top of each plot. The shaded ranges correspond to the 25–75% quartiles with the median indicated separately (analogous to a common boxplot). The violin plots show that NEU4 is induced in carriers of allele T on LPS exposure, whereas NEU4 expression is reduced in homozygotes of allele C. Full size image SNP rs1719126 on chromosome 17q12 is the most significant trans iQTL and additionally represents the third strongest cis iQTL ( Supplementary Table 1 ). In cis rs1719126 regulates the expression of the chemokine (C-C motif) ligand 14 ( CCL14 ) gene, whose transcription start site (TSS) is 101 kb distant from rs1719126 ( P LPS =5.80 × 10 –30 , Fig. 3a ). Chip-seq data from ENCODE [13] revealed an RNA polymerase II binding site overlapping rs1719126, which represents a potential mechanism of CCL14 regulation ( Supplementary Fig. 6 ). On the functional level, CCL14 is a highly expressed chemokine, whose activity as a chemotactic signal for pro-inflammatory cells is mainly regulated by a proteolytic processing step [14] . Our data now reveal that CCL14 is additionally regulated at the transcriptional level with strong genetic determination. 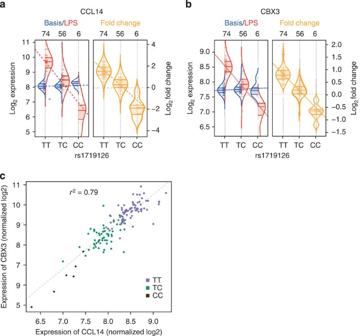Figure 3: rs1719126 represents the strongesttransand the third strongestcisiQTL during TLR4 signalling. (a) In homozygous carriers of allele T,CCL14expression is induced on LPS exposure and reduced in homozygotes for the opposite allele. (b) The allele-specific expression ofCBX3is nearly identical to that observed forCCL14. The same homozygous T carriers show an induction ofCBX3expression on LPS exposure, whereas a reduced expression is observed in homozygotes for the opposite allele. (c) Correlation ofCCL14andCBX3expressions on LPS exposure (r2=0.79).Violin plots are depicted as inFig. 2. Figure 3: rs1719126 represents the strongest trans and the third strongest cis iQTL during TLR4 signalling. ( a ) In homozygous carriers of allele T, CCL14 expression is induced on LPS exposure and reduced in homozygotes for the opposite allele. ( b ) The allele-specific expression of CBX3 is nearly identical to that observed for CCL14 . The same homozygous T carriers show an induction of CBX3 expression on LPS exposure, whereas a reduced expression is observed in homozygotes for the opposite allele. ( c ) Correlation of CCL14 and CBX3 expressions on LPS exposure ( r 2 =0.79).Violin plots are depicted as in Fig. 2 . Full size image In trans rs1719126 regulates the expression of the chromobox protein homolog 3 ( CBX3 ) gene on chromosome 7p15 ( P LPS =3.48 × 10 –28 , Fig. 3b ). We observed a strong correlation between CCL14 and CBX3 expressions among our volunteers ( r 2 =0.79, Fig. 3c ), indicating that cis -modulation of CCL14 results in differential expression of CBX3 . While previous studies have found that CBX3 acts as a heterochromatin protein [15] , a recent study has shown that CBX3 directly regulates the expression and splicing of many genes [16] . In particular, after cytokine exposure CBX3 is specifically recruited to inflammatory genes [16] . Next, we used differential gene expression on TLR4 stimulation (ΔLPS/baseline) as an alternative quantitative trait to identify iQTLs that are already present in unstimulated monocytes but have additional allele-specific effects during immune response ( Supplementary Fig. 4 ). Among these, rs10239340 on chromosome 7q32 acts in cis on the expression of interferon 5 ( IRF5 ) and represents the most significant iQTL ( Supplementary Table 2 ). In baseline monocytes, carriers of the T allele show elevated IRF5 expression compared with carriers of the opposite allele ( P Baseline =3.97 × 10 –59 ). However, on TLR4 stimulation T-allele carriers show an allele-specific downregulation of IRF5 ( P ΔLPS/Baseline =1.63 × 10 –35 , Fig. 4 ). IRF5 represents a key pro-inflammatory transcription factor for the expression of many immune-relevant genes [17] . Thus, IRF5 expression differences during TLR4 signalling probably affect pro-inflammatory immune response at later time points. 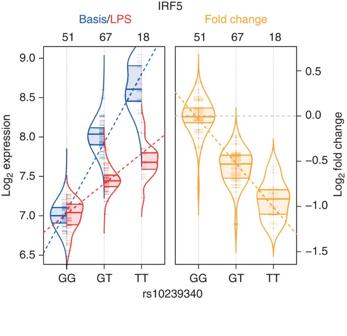Figure 4: rs10239340 represents the strongest iQTL during TLR4 signalling that is also functionally active in baseline monocytes and shows an additional regulatory effect on differential expression on LPS exposure. Carriers of the T allele have elevated baselineIRF5expression compared with individuals carrying the G allele (left; blue violin plots). On LPS exposure a robust downregulation ofIRF5proportional to the number of T alleles is observed, whereas no differential regulation is seen in homozygotes for the G allele (right; orange violin plots). Violin plots are depicted as inFig. 2. Figure 4: rs10239340 represents the strongest iQTL during TLR4 signalling that is also functionally active in baseline monocytes and shows an additional regulatory effect on differential expression on LPS exposure. Carriers of the T allele have elevated baseline IRF5 expression compared with individuals carrying the G allele (left; blue violin plots). On LPS exposure a robust downregulation of IRF5 proportional to the number of T alleles is observed, whereas no differential regulation is seen in homozygotes for the G allele (right; orange violin plots). Violin plots are depicted as in Fig. 2 . Full size image eQTLs for the expression of IRF5 have been previously found in unstimulated LCLs and whole-blood samples [18] , [19] . In LCLs we observed an opposing directional eQTL effect [18] compared with monocytes. Here, carriers of the G allele showed elevated IRF5 expression compared with carriers of allele T. In contrast, in whole-blood samples [19] we studied rs10229001, which is in perfect LD to our eQTL marker ( r 2 =1) and observed the same expression effect as seen in monocytes. Thus—besides the context specific eQTL effect on LPS stimulation—rs10239340 represents a cell-type-specific eQTL. Recently lysozyme ( LYZ ) on chromosome 12q15 has been described as a monocyte-specific master regulator eQTL [20] . In this study, rs10784774 was identified as cis eQTL for LYZ and as trans eQTL for 62 other genes under baseline condition. Analysis of hotspots in our data confirms LYZ as a master regulator ( Supplementary Fig. 7a ). LYZ was allele-specifically regulated in cis ( P Baseline =4.38 × 10 –37 ) and a total of 108 different genes in trans ( Supplementary Fig. 7b and Supplementary Data 7 ). This master regulator eQTL was also present in stimulated monocytes ( Supplementary Fig. 7 ). However, no LYZ -regulated transcript showed a significant differential expression on TLR4 stimulation, indicating that this pathway does not play a prominent role in the early phase of TLR4 signalling. Finally, we tested whether SNPs that have been identified as risk factors for common diseases represent iQTLs and used all SNPs that have been deposited in the Catalog of Published Genome-Wide Association Studies. This revealed many GWAS-SNPs that are eQTLs under baseline and TLR4-signalling condition ( Supplementary Data 8 ) as well as GWAS-SNPs as being active iQTLs only during TLR4 signalling. The most significant GWAS-iQTL represents rs968451 on chromosome 22q13, which regulates the expression of the platelet-derived growth factor beta polypeptide ( PDGFB ) gene in cis . The expression of PDGFB is induced during TLR4 signalling strongest for carriers of the common allele G ( P LPS =4.31 × 10 –12 , P ΔLPS/Baseline =6.09 × 10 –12 , Fig. 5a ). SNP rs968451 is located 30 kb distant to the TSS of PDGFB and also confers risk for primary biliary cirrhosis (PBC) [21] , a severe autoimmune liver disease characterized by a destructive cholangitis. In this GWAS, the authors favoured MAP3K7IP1 as being the risk-conferring PBC gene at this locus [21] , which is located 125 kb distant to rs968451. However, the testing of all transcripts within a 10-Mb interval of rs968451 in our data set revealed that PDGFB is the only transcript regulated by the PBC risk variant during TLR4 signalling ( Fig. 5b ). 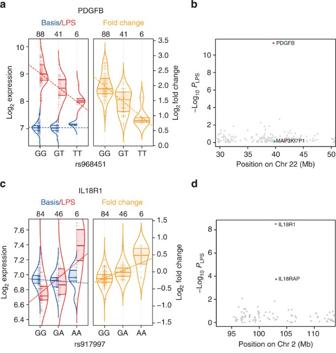Figure 5: rs968451 and rs917997 represent the strongest GWAS-iQTL during TLR4 signalling. (a)PDGFBexpression is allele-specifically induced on LPS exposure, strongest for carriers of allele G. Violin plots are depicted as inFig. 2. (b) Regional association plot from stimulated monocytes shows that rs968451 regulatesPDGFBexpression selectively (red dot). In particular,MAP3K7IP1expression is not allele-specifically influenced by rs968451 (green dot). (c) In homozygous A carriers,IL18R1expression is induced on LPS exposure and reduced in G carriers. Violin plots are depicted as inFig. 2. (d) Regional association plot from stimulated monocytes shows that rs917997 regulatesIL18R1expression strongest (red dot). In particular the expression of genes belonging to the interleukin receptor cluster are not allele-specifically influenced by rs917997, althoughIL18RAPshows a tendency towards iQTL-regulation (PLPS=1.8 × 10−4, green dot). Figure 5: rs968451 and rs917997 represent the strongest GWAS-iQTL during TLR4 signalling. ( a ) PDGFB expression is allele-specifically induced on LPS exposure, strongest for carriers of allele G. Violin plots are depicted as in Fig. 2 . ( b ) Regional association plot from stimulated monocytes shows that rs968451 regulates PDGFB expression selectively (red dot). In particular, MAP3K7IP1 expression is not allele-specifically influenced by rs968451 (green dot). ( c ) In homozygous A carriers, IL18R1 expression is induced on LPS exposure and reduced in G carriers. Violin plots are depicted as in Fig. 2 . ( d ) Regional association plot from stimulated monocytes shows that rs917997 regulates IL18R1 expression strongest (red dot). In particular the expression of genes belonging to the interleukin receptor cluster are not allele-specifically influenced by rs917997, although IL18RAP shows a tendency towards iQTL-regulation ( P LPS =1.8 × 10 −4 , green dot). Full size image Our data show that the PBC variant rs968451 regulates PDGFB expression with reduced transcript levels in risk allele carriers. This function is only active during TLR4 signalling, which fits pathophysiological concepts, according to which TLR signalling confers PBC risk [22] . We therefore suggest PDGFB as a novel PBC risk gene at this locus. Also, on the functional level PDGFB represents a plausible PBC risk gene, given its involvement in the induction of angiogenesis, a process that has been linked to the pathophysiology of PBC [23] . The second GWAS-iQTL concerns rs917997 on chromosome 2q12, which is 91 kb distant to the TSS of the interleukin 18 receptor 1 ( IL18R1 ) gene and regulates its expression in cis . Only during TLR4 signalling is the expression of IL18R1 induced in homozygous A carriers and reduced in homozygous carriers of the opposite allele ( P LPS =3.10 × 10 –9 , P ΔLPS/baseline =5.99 × 10 –11 , Fig. 5c ). Allele A of rs917997 has been identified as a risk factor for inflammatory bowel disease (IBD) [24] and celiac disease [25] , both inflammatory diseases of the intestine. However, based on GWAS data it was not possible to favour a risk gene, because IL18R1 forms, together with the interleukin receptor genes IL1R1 , IL1R2 , IL1RL1, IL1RL2 and IL18RAP , a cluster at this locus. We tested whether these or other nearby genes are also regulated by rs917997 during TLR4 signalling. Although not significant, IL18RAP is additionally cis -regulated within a 10-Mb interval of the risk variant ( P LPS =1.8 × 10 –4 , Fig. 5d and Supplementary Fig. 8 ). Our data show that rs917997 becomes functionally active only during TLR4 signalling and thereby influences IL18R1 expression and to lesser extent IL18RAP expression. IL18R1 and IL18RAP form the heterodimeric IL18 receptor complex, which relays IL18-dependent signal transduction to the NFκB-pathway [26] . As such, IL18R1 and IL18RAP represent plausible risk genes for IBD and celiac disease at this locus, particularly as alterations in IL18- and TLR-mediated processes have been reported for both disorders [27] . As for IRF5 , an eQTL effect of rs917997 on the expression of IL18RAP has been previously described in unstimulated whole-blood samples [28] . In this study, opposing directional expression effects compared with monocytes have been observed. Carriers of allele G show elevated IL18RAP expression levels compared with carriers of allele A. This further exemplifies that gene regulation represents a complex cell–type- and context-specific process. Whether cell-type-specific eQTLs are functionally more susceptible to environmental influences, such as exogenous cell stimulation, represents an interesting hypothesis. However, future studies could test this hypothesis, as eQTL data for large numbers of different cell types become increasingly available. Recently two studies identified eQTLs under LPS stimulation in primary human monocytes [29] and dendritic cells [30] . Comparison of our study with these studies showed a significant overlap between our data and those of Fairfax et al. [29] In all, 43 and 44% of our monocyte data under baseline and LPS stimulation, respectively, were found to be genome-wide significant in Fairfax et al. ( Supplementary Fig. 9a ) and 55 (baseline) and 56% (LPS) of the data of Fairfax et al. showed evidence of replication in our data set ( Supplementary Fig. 9b ). Lee et al. [30] used a targeted approach (415-gene signature) to identify LPS-responsive eQTLs after 5-h LPS treatment in dendritic cells and showed little overlap with both monocytes works, which, however, can be explained by differences in experimental design ( Supplementary Fig. 9a and b ). To discover further immune-relevant eQTLs that might have been missed due to limited power, we performed a replication analysis using data from Fairfax et al. [29] This led to the identification of 672 cis and 237 trans additional iQTLs unique to TLR4 stimulation under absolute expression and 222 cis and 79 trans additional iQTLs under differential expression ( Supplementary Fig. 9c and Supplementary Data 3–5 ). Taken together, this demonstrates the robustness of identifying immune-relevant eQTLs on LPS stimulation. In summary, eQTL studies in the context of cellular LPS exposure provide comprehensive insights into the genetic regulation of innate immunity. Among these, functional SNPs for the expression of NEU4 , CCL14 , CBX3 and IRF5 contributed strongest to interindividual differences in immune response. Furthermore, we found that risk variants for PBC, IBD and celiac disease exclusively regulate the expression of PDGFB and IL18R1 during immune response. Both genes are plausible candidates to study the disease pathophysiology in context of immune activation. Of course, follow-up studies on the biological function of the here identified eQTLs will be essential to gain further insights into the mechanisms of genetic variants regulating innate immune responses. Our study represents an innovative approach to gain insights into gene–environmental interactions. The use of exogenous cell stimulation followed by eQTL identification might contribute to the elucidation of the physiology and pathophysiology of many cellular processes and diseases. Sample collection, isolation and stimulation of CD14+ monocytes In total, 185 healthy male volunteers of German descent were recruited. The study was approved by the institutional review board of the University of Bonn. All volunteers signed informed consent and were between age 18 and 35 (mean 24). PBMC were obtained by Ficoll-Hypaque density gradient centrifugation of heparinized blood. Monocytes were isolated with anti-CD14 para-magnetic beads according to the manufacturer’s manual (MACS, Miltenyi Biotec). The purity of isolated monocytes was ≥95%. RPMI 1640 (Biochrom) supplemented with 10% heat-inactivated FCS (Invitrogen), 1.5 mM L -glutamine, 100 U ml −1 penicillin, 100 μg ml −1 streptomycin (all Sigma-Aldrich) and 10 ng ml −1 GM-CSF (ImmunoTools) was used to culture cells in 96-well round bottom wells at a density of 250,000 cells per well in 100 μl overnight. Cell survival after overnight incubation was >85%. Cells of each volunteer were either untreated or treated with 200 ng ml −1 ultrapure LPS from Escherichia coli (Invivogen). After 90 min cells were lysed in RLT reagent (Qiagen) and stored at −80 °C. C-reactive protein (CRP) levels were measured to exclude samples with elevated CRP levels. After stringent quality control (Non-smoker, no infection or vaccination 4 weeks before blood withdrawal, CRP <2.5 mg dl −1 , monocyte purity ≥95%, monocyte survival >85%), final samples from 137 individuals were further processed. RNA extraction RNA was extracted from the lysed cells using the AllPrep 96 DNA/RNA Kit from Qiagen. RNA concentrations were determined using NanoDrop (PeqLab) and a subset of samples was additionally checked for degradation in a Bioanalyser (Agilent Technologies). Gene expression analysis The Illumina TotalPrep-96 RNA Amplification Kit (Life Technologies) was used for the amplification and biotinylation of the RNA. Subsequent array-based gene expression analysis was performed on Illumina’s Human HT-12 v4 Expression BeadChips (Illumina) comprising 47,231 probes. Expression profiles were normalized using function vsn2 implemented in the Bioconductor package ‘vsn’ [31] . Only probes that showed a P detection <0.01 in more than 5% of at least one of the two conditions (baseline, LPS) were analysed. Probes that matched to multiple positions in the human genome and probes mapping to non-autosomal chromosomes were excluded from further analysis. Finally, probes were removed if SNPs within a probe showed an eQTL effect to the respective gene, resulting in 17,684 probes for statistical analyses. DNA extraction Genomic DNA was extracted from 10 ml blood using the Chemagic Magnetic Separation Module I (PerkinElmer Chemagen) according to the manufacturer’s instructions. DNA was quantified by NanoDrop (PeqLab). DNA genotyping Genotyping was conducted on the Illumina’s HumanOmniExpress BeadChips comprising 730,525 SNPs. After quality control ( P HWE >10 –5 , call rate >98%, MAF >5%), a total of 579,090 SNPs were available for analysis. Samples showing potential admixture within the multi-dimensional scaling analysis were removed. All samples showed a call rate >99%. SNP imputation of GWAS findings SNPs reported in previous GWAS and not present on the HumanOmniExpress BeadChips were imputed. Imputation was performed using IMPUTE2 (ref. 32 ) based on 1,000 Genomes Pilot I (European) as a reference panel. Pathway analysis Data were evaluated using Ingenuity Pathway Analysis (IPA; Ingenuity Systems, Redwood City, CA, USA). IPA maps each gene within a global molecular network developed from information contained in the Ingenuity Pathways Knowledge Base. Gene networks were generated algorithmically based on their connectivity in terms of expression, activation and transcription. A ‘network’ in IPA is defined as a graphical representation of the molecular relationships between genes, which are represented as nodes, and the biological relationship between nodes is shown by a connecting line. All connections are supported by published data stored in the Ingenuity Pathways Knowledge Base and/or PubMed [33] . Pathway enrichment analysis of differentially expressed genes, clusters of co-correlated genes and eQTL genes was performed using InnateDB [34] . eQTL-analysis Association tests were corrected for the top 10 multi-dimensional scaling components. As phenotypes, we mapped absolute expression values of untreated ( P Baseline ), LPS-treated ( P LPS ) and the differential expression of LPS-treated monocytes ( P ΔLPS/Baseline ) separately. Association between SNP genotypes and gene expression levels was examined by using a linear regression model of the phenotype versus minor allele dosage of the genotype (additive model). All possible SNP/phenotype combinations were tested exhaustively using PLINK v1.07 (ref. 35 ), downstream analyses were carried out using R with appropriate packages and in-house codes. cis -acting eQTLs were defined as SNPs located within 1-Mb interval on either side of a transcript to differentiate them from trans -acting eQTLs. MANOVA implemented in R was used to map shared eQTLs between treated and untreated monocytes, which is equivalent to the Bayesian formulation given in a previous study [7] . P LPS and P Baseline from standard univariate analysis were compared with P Manova . This revealed 3,154 genome-wide significant eQTLs (corresponding to 690 genes) at P Manova <1.76 × 10 –09 with an FDR of 0.01 where P Manova <min( P LPS, P Baseline ) and P Baseline <8.67 × 10 –09 and P LPS <7.35 × 10 –09 . Replication of eQTLs The study data set was compared with a recently published eQTL data set under LPS stimulation [29] , which used the same Illumina HumanHT-12 expression and HumanOmniExpress genotyping platform. We conducted a replication analysis of peak cis eQTLs (6,509 eQTLs under baseline and 6,513 eQTLs on 2-h LPS stimulation) from Fairfax et al. [29] This revealed (i) 1,731 additional cis eQTLs under baseline condition (corresponding to 1,092 genes; P Baseline.cis <4.15 × 10 −03 , FDR of 0.01), (ii) 1,659 cis eQTLs on LPS stimulation (corresponding to 1,083 genes; P LPS.cis <3.87 × 10 −03 , FDR of 0.01) and (iii) 222 cis iQTLs when fold change on LPS treatment is considered (corresponding to 161 genes; P ΔLPS/Baseline cis <3.5 × 10 −04 , FDR of 0.01). Testing trans eQTLs (4,354 eQTLs under baseline and 2,359 eQTLs on 2-h LPS stimulation) of the same study revealed (iv) 1,671 additional trans eQTLs under baseline condition (corresponding to 137 genes; P Baseline.trans <5.82 × 10 −03 , FDR of 0.01), ( v ) 1,050 trans eQTLs on LPS stimulation (corresponding to 109 genes; P LPS.trans <7.32 × 10 −03 , FDR of 0.01) and ( vi ) 79 trans iQTLs when fold change on LPS treatment is considered (corresponding to 14 genes; P ΔLPS/Baseline trans <1.71 × 10 −04 , FDR of 0.01). Replication analysis of P Baseline and P LPS were conducted on a per-condition basis with identical effect directions, whereas for P ΔLPS/baseline the union of eQTLs under baseline and LPS treatment was used. For the latter, we checked for identical effect directions in both the treated and untreated conditions. How to cite this article: Kim, S. et al. Characterizing the genetic basis of innate immune response in TLR4-activated human monocytes. Nat. Commun. 5:5236 doi: 10.1038/ncomms6236 (2014).